Dirac cones and Dirac saddle points of bright excitons in monolayer transition metal dichalcogenides In monolayer transition metal dichalcogenides, tightly bound excitons have been discovered with a valley pseudospin optically addressable through polarization selection rules. Here, we show that this valley pseudospin is strongly coupled to the exciton centre-of-mass motion through electron-hole exchange. This coupling realizes a massless Dirac cone with chirality index I =2 for excitons inside the light cone, that is, bright excitons. Under moderate strain, the I =2 Dirac cone splits into two degenerate I =1 Dirac cones, and saddle points with a linear Dirac spectrum emerge. After binding an extra electron, the charged exciton becomes a massive Dirac particle associated with a large valley Hall effect protected from intervalley scattering. Our results point to unique opportunities to study Dirac physics, with exciton’s optical addressability at specifiable momentum, energy and pseudospin. The strain-tunable valley-orbit coupling also implies new structures of exciton condensates, new functionalities of excitonic circuits and mechanical control of valley pseudospin. The strong coupling of an internal degree of freedom with motion can give rise to quasiparticles with radically new behaviours. A seminal example is the Dirac cones in graphene and topological insulators where low-energy carriers are found with linear dispersion and spin-momentum locking [1] , [2] , [3] , [4] . These massless Dirac fermions are drawing great interest for their scientific and technological importance. Besides the Dirac cone, other band geometries exhibiting a linearly dispersing Dirac spectrum are being discovered including the Dirac circle and Dirac arc [5] , the Dirac node [6] , the anisotropic Dirac cone [7] and the three-dimensional Dirac point [8] . The interest on Dirac particles also drives the extensive efforts to realize Dirac spectra by engineering artificial honeycomb lattices of electrons, atoms and photons [9] , [10] , [11] . An exciton is a composite particle comprising of an electron and a hole in hydrogen-like bound state, which plays key roles in optoelectronic phenomena and applications. An exciton can be interconverted with a photon under the constraint of energy–momentum conservation. In two-dimensional (2D) systems, this coupling to photons makes possible the optical preparation of exciton at any specified energy ( E ) and wavevector ( k ) on its dispersion in the light cone (the conical region defined by E ≥ ħc | k |), as well as the optical detection for mapping out the distribution of such bright excitons in energy–momentum space [10] , [11] . In semiconductors, the bright excitons can have lifetimes long enough to allow for the formation of an exciton condensate [12] , [13] , and controlled flow in an integrated excitonic circuit [14] . Monolayer group-VIB transition metal dichalcogenides (TMDCs) offer a new 2D material system to explore exciton physics. These are direct bandgap semiconductors, with the conduction and valence band edges at the doubly degenerate corners (± K points) of the hexagonal Brillouin zone [15] , [16] . The bright exciton thus has two valley pseudospin configurations where the electron and hole are both confined at either the K or − K valley [17] . An optical selection rule dictates that an exciton in these two valley states couples respectively to a σ + or σ − circularly polarized photon only [18] , which makes possible optical generation of excitonic valley polarization and coherence as demonstrated recently [19] , [20] , [21] , [22] . Moreover, the Coulomb interaction between the electron and hole is exceptionally strong due to their heavy masses and the 2D confinement. Sharp exciton and trion resonances are seen in the photoluminescence (PL) spectrum with a charging energy of ∼ 30 meV (refs 22 , 23 , 24 ), compatible with the exciton binding energy of ∼ 0.5–1 eV from ab initio calculations [17] , [25] , [26] , [27] , [28] . Here we show that in monolayer TMDC, the pronounced electron-hole Coulomb exchange in exciton realizes a strong valley-orbital coupling that can be orders of magnitude larger than the radiative recombination and momentum scattering rates. In such a strong coupling regime, the pseudospin splitting from the valley-orbit coupling becomes spectrally resolvable. A bright exciton in the light cone thus behaves like a massless Dirac particle, where the in-plane rotation symmetry dictates that it must have chirality index ( I ) of 2 (that is, the valley pseudospin rotates 4 π when momentum circles the Dirac point once), distinct from all known Dirac particles. Moderate tensile strain can realize a sizable in-plane Zeeman field on the exciton valley pseudospin, which splits the I =2 Dirac cone into two degenerate I =1 cones centred at opposite momentums. Consequently, a new type of band geometry, the linearly dispersing Dirac saddle points, emerges in the light cone. When the exciton binds an electron to form a trion, the exchange interaction with the excess electron opens up a gap at the Dirac point, turning the trion into a massive Dirac particle associated with a large valley Hall effect protected from intervalley scattering. Massless Dirac cone of bright exciton The bright exciton X 0 in the two valley configurations is schematically shown in Fig. 1a . The valence band has a large valley-dependent spin splitting of ∼ 150–450 meV (refs 18 , 29 ). The spin index of the band edge hole states are therefore locked with the valley index, that is, K (− K ) valley has spin up (down) states only. Spin is unchanged by the optical transition, leaving only two possible configurations for bright exciton. We use to denote the exciton valley pseudospin, where pseudospin-up (down) corresponds to X 0 at the K (− K ) valley that couples to a σ+ (σ−) photon only. X 0 with an in-plane pseudospin, that is, a superposition of the two valley configurations, then couples to a linearly polarized photon. 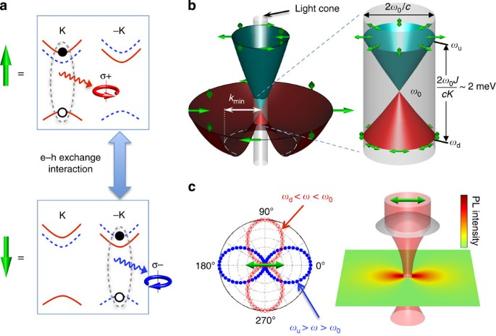Figure 1: Valley-orbit coupled neutral exciton X0. (a) Valley pseudospin-up and -down configurations of X0, which recombine to emitσ+ andσ− photon respectively. Red (blue) lines denotes spin up (down) conduction and valence band edges inKand −Kvalleys, and solid (hollow) circle denotes the electron (hole). Electron-hole exchange interaction acts as an in-plane field that couples the two valley configurations depending on the exciton centre-of-mass wavevectork. The conduction band spin splitting of WX2(X=S, Se) is shown here, while the valley-orbit coupling of bright exciton is independent of this spin splitting and is present for both WX2and MoX2. (b) Dispersion of valley-orbit coupled X0, which, in the light cone, realizes a massless Dirac cone with chirality indexI=2. The single-head arrows denote the valley pseudospin at variousk. In the zoom-in of the dispersion in the light cone, double-head arrows are used to denote the linear polarization of the emitted photon upon exciton recombination. (c) Schematic setup for observing spin-momentum locking of X0. Blue (red) dots in the polar plot denote the angular distribution of X0ink-space when the upper (lower) branch of Dirac cone is resonantly excited by a linearly polarized laser with a diffraction-limited beam focus. Ballistic transport converts this distribution ink-space into the same angular distribution in real space for observation. Figure 1: Valley-orbit coupled neutral exciton X 0 . ( a ) Valley pseudospin-up and -down configurations of X 0 , which recombine to emit σ + and σ − photon respectively. Red (blue) lines denotes spin up (down) conduction and valence band edges in K and − K valleys, and solid (hollow) circle denotes the electron (hole). Electron-hole exchange interaction acts as an in-plane field that couples the two valley configurations depending on the exciton centre-of-mass wavevector k . The conduction band spin splitting of WX 2 (X=S, Se) is shown here, while the valley-orbit coupling of bright exciton is independent of this spin splitting and is present for both WX 2 and MoX 2 . ( b ) Dispersion of valley-orbit coupled X 0 , which, in the light cone, realizes a massless Dirac cone with chirality index I =2. The single-head arrows denote the valley pseudospin at various k . In the zoom-in of the dispersion in the light cone, double-head arrows are used to denote the linear polarization of the emitted photon upon exciton recombination. ( c ) Schematic setup for observing spin-momentum locking of X 0 . Blue (red) dots in the polar plot denote the angular distribution of X 0 in k -space when the upper (lower) branch of Dirac cone is resonantly excited by a linearly polarized laser with a diffraction-limited beam focus. Ballistic transport converts this distribution in k -space into the same angular distribution in real space for observation. Full size image The Coulomb exchange interaction between the electron and hole of X 0 will couple its two valley configurations, giving rise to an effective interaction between the exciton’s centre-of-mass momentum k =( k cos θ , k sin θ ) and its valley pseudospin (see Supplementary Note 1 ). The valley-orbit coupling is of the form: J ( k )= j ( k ) e −2 i θ , where the strength of the coupling . Here, a is the lattice constant, E g the bandgap and t is the nearest neighbour hopping integral in the monolayer TMDCs [18] . V ( k ) is the Fourier transform of the Coulomb interaction, and is the wavefunction of the electron-hole relative motion. thus corresponds to the probability of finding the electron and hole spatially overlapped. where a B is the Bohr radius. By this effective valley-orbit coupling, the exciton dispersion splits into two branches with energies (see Fig. 1b ), where ħ ω 0 , the exciton energy at k =0, is about 2 eV (refs 22 , 23 , 24 ), and M 0 , the exciton mass, is about the same as the free electron mass. Each branch has a I =2, that is, the valley pseudospin lies in the plane and rotates twice when the momentum undergoes one full circle around k =0. This pseudospin chirality is dictated by the in-plane rotation symmetry of the lattice and the optical polarization selection rule associated with the exciton valley pseudospin. A photon emitted by the upper (lower) branch is linearly polarized with the projection of the polarization vector in the 2D plane being longitudinal (transverse) to the momentum k . Such a longitudinal-transverse splitting is known in GaAs quantum wells [30] , where it can give rise to exciton spin relaxation [31] and the optical spin Hall effect [32] . However, two features distinguish this effect in monolayer TMDCs. First, the exciton eigenstates are now coherent superpositions at two well-separated valleys in momentum space, where the splitting corresponds to a Rabi oscillation between the two valleys. Second, the magnitude of the splitting can be orders larger in TMDC monolayers than that in a GaAs quantum well, due to the much stronger Coulomb binding (represented by ) (refs 23 , 24 , 25 ). The Coulomb interaction in an intrinsic 2D semiconductor is of the unscreened form: (ref. 30 ). Thus, the valley-orbit coupling strength scales linearly with the momentum k : , where . is the distance from the ± K points to the Γ point of the Brillouin zone. We note that corresponds to the exciton binding energy which in monolayer TMDCs is ∼ 0.5–1 eV (refs 17 , 23 , 24 , 25 ), more than one order of magnitude larger than that in GaAs quantum wells. Ab initio calculations also find the exciton Bohr radius a B ∼ 1 nm (refs 17 , 24 , 25 , 33 ), one order of magnitude smaller than that in GaAs. Thus, the splitting in monolayer TMDCs is two orders of magnitude stronger than that in GaAs quantum wells. With the parameters a , E g and t from band structure calculations [18] , we estimate J ∼ 1 eV. Because of the strong valley-orbit coupling, the energy minimum of the exciton dispersion appears on a ring with radius k min ∼ 0.05 K , which is outside the light cone defined by | k |≤ω 0 / c ∼ 10 −3 K (c.f. Fig. 1b ). At the light cone edge, the valley pseudospin splitting , well exceeding the exciton’s radiative decay rate and momentum scattering rate expected in clean samples at low temperature [13] , [19] , [34] . Thus, in the light cone, the exciton has a conical dispersion that can be spectrally resolved. The bright exciton behaves effectively like a massless Dirac particle, with an I =2 and a group velocity J / ħK ∼ 10 5 m s −1 . These are in sharp contrast to GaAs quantum wells, where the longitudinal-transverse splitting cannot be spectrally resolved [30] , [31] . The optical addressability of bright excitons provides unique opportunities to investigate Dirac particles. As an example, Fig. 1c schematically illustrates a setup for the direct observation of spin-momentum locking of massless Dirac particle. Using laser pulses with a narrow frequency and diffraction-limited beam spot, we can resonantly excite excitons, selectively on an energy contour in the upper or lower branch of the Dirac cone. By using linearly polarized excitation [22] , the population distribution of injected excitons is anisotropic in momentum space with the angular dependence of ∝ cos 2 θ ( ∝ sin 2 θ ) if the upper (lower) branch is on resonance (c.f. Fig. 1c ). Ballistic propagation will convert this angular distribution in momentum space into the same angular distribution in real space, which may be observed from the spatial map of the PL. Effects of strain on bright exciton and the Dirac saddle points The electron-hole exchange also realizes the coupling between exciton valley pseudospin and mechanical strain. Due to rotational symmetry of the monolayer TMDCs, the valley pseudospin splitting must vanish at k =0. However, an in-plane uniaxial tensile strain [35] , [36] , [37] that breaks the rotational symmetry can introduce a finite splitting at k =0. Our ab initio calculation on monolayer WSe 2 shows that the strain realizes an in-plane Zeeman field on the valley pseudospin (see Supplementary Note 2 ), and the exciton Hamiltonian becomes For strain applied along the armchair ( x ) and zigzag ( y ) directions (see Fig. 2 ), we find J 0 along the positive x -axis and the negative x -axis respectively. Its magnitude as function of the strain strength is shown in Fig. 2c . A moderate strain of 1% can already induce a valley pseudospin splitting of ∼ 12 meV, spectrally resolvable with existing sample qualities [22] . 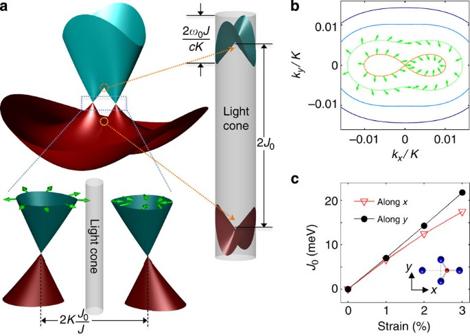Figure 2: Strain effect on X0. (a) The strain acts as an in-plane Zeeman fieldJ0on valley pseudospin, splitting the single Dirac cone of chirality indexI=2 into two Dirac cones ofI=1. Consequently, two Dirac saddle points of linear dispersion appear in the light cone. (b) Contour plot of the higher energy branch. The green arrows illustrate the valley pseudospin configurations. (c) The calculated magnitude ofJ0as a function of the strength of strain applied along thexandydirections shown in the inset (seeSupplementary Note 2). Figure 2: Strain effect on X 0 . ( a ) The strain acts as an in-plane Zeeman field J 0 on valley pseudospin, splitting the single Dirac cone of chirality index I =2 into two Dirac cones of I =1. Consequently, two Dirac saddle points of linear dispersion appear in the light cone. ( b ) Contour plot of the higher energy branch. The green arrows illustrate the valley pseudospin configurations. ( c ) The calculated magnitude of J 0 as a function of the strength of strain applied along the x and y directions shown in the inset (see Supplementary Note 2 ). Full size image The strain effect makes possible a controllable way to coherently rotate the exciton valley pseudospin at k =0. An even more interesting consequence is the Dirac cone with I =2 now splits into two Dirac cones with I =1 each, as shown in Fig. 2 . From equation (1), the two new Dirac points are , θ 0 being the direction angle of J 0 . With a strain of 1%, both new Dirac points are well outside the light cone. The two new Dirac cones are anisotropic, with the velocity in the armchair direction being half of that in the zigzag direction. In the light cone, the two Dirac cones merge in the form of saddle points in both the upper and lower branches of the dispersion. Remarkably, the saddle points are linearly dispersed along all directions. Such Dirac type saddle points are unique to excitons in monolayer TMDCs and have not been discussed in any system. This is a generic consequence when a Dirac cone of I =2 is subject to an in-plane Zeeman field on the pseudospin. Gapped Dirac cone and valley Hall effect of negative trion Now we turn to negatively charged trion X– where an electron-hole pair binds an excess electron. Interestingly, the Coulomb exchange with the excess electron opens up a gap at the excitonic Dirac point, turning trion into a massive Dirac particle associated with a large Berry curvature. We note that conduction band edges in the ± K valleys also feature a valley-dependent spin splitting. The size of the splitting ranges from several to several tens of meV, and there is an overall sign difference between molybdenum dichalcogenides and tungsten dichalcogenides [29] . Below, we consider monolayer WX 2 (X=S, Se) only, where the spin splitting ∼ 30 meV and the spin configurations of the conduction band edges in the ± K valleys are schematically shown in Fig. 1a . X– has four ground state configurations that can recombine to emit photon, as shown in Fig. 3a . With the ∼ 30 meV conduction band spin splitting, the excess electron is in the lowest energy band where optical transition to the valence band edge is spin forbidden. With the excess electron in the K (− K ) valley, X– has the centre-of-mass wavevector q X− ≡K + k ( q X− ≡−K+k ). In principle, X– with any k can recombine as the recoil of the excess electron can facilitate the momentum conservation, but the recombination rate decays here as ∼ exp(− k 2 /(0.01 K ) 2 ), [24] which we define as the trion brightness. Trion emission is thus expected mainly in the region k ≲ 0.01 K . 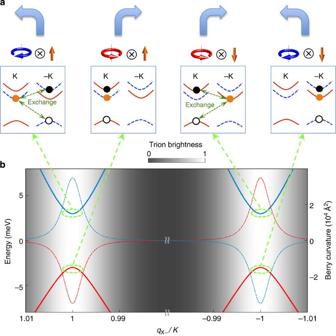Figure 3: Massive Dirac cones of negatively charged trion X–. (a) The four configurations of X– that can emit photons in monolayer WX2, labelled by the spin of the excess electron and polarization of the photon emission. The latter is determined by the valley pseudospin of the electron-hole pair that can recombine (black circles). (b) The solid lines plot the dispersion of X–, where a gap is opened at the Dirac points by the exchange coupling of the electron-hole pair with the excess electron. Whiteness of the background corresponds to the brightness of X– as function of center-of-mass wavevectorqX−. The blue (red) dashed lines plot the Berry curvature of the upper (lower) branch of the dispersion, which gives rise to the anomalous transverse motion of X– in an electric field, as illustrated by curved arrows ina. Figure 3: Massive Dirac cones of negatively charged trion X–. ( a ) The four configurations of X– that can emit photons in monolayer WX 2 , labelled by the spin of the excess electron and polarization of the photon emission. The latter is determined by the valley pseudospin of the electron-hole pair that can recombine (black circles). ( b ) The solid lines plot the dispersion of X–, where a gap is opened at the Dirac points by the exchange coupling of the electron-hole pair with the excess electron. Whiteness of the background corresponds to the brightness of X– as function of center-of-mass wavevector q X− . The blue (red) dashed lines plot the Berry curvature of the upper (lower) branch of the dispersion, which gives rise to the anomalous transverse motion of X– in an electric field, as illustrated by curved arrows in a . Full size image The four X– configurations can be distinguished by : the valley index of the electron-hole pair that can recombine, and : the spin index of the excess electron. The former is associated with the circular polarization of the emitted photon. Like X 0 , the exchange interaction between the pair of electron and hole in the same valley with opposite spin will couple the two valley configurations with identical . Due to the rotational symmetry of the lattice, the coupling is still of the form , where k =( k cos θ , k sin θ ). The coupling strength J is about the same to that in the X 0 case. In addition, there is also exchange interaction between the excess electron with the electron-hole pair ( Fig. 3 ), which only affects the two X– configurations where and have the same sign (first and third one in Fig. 3a ) and raises their energy by an amount estimated to be δ ∼ 6 meV (see Supplementary Note 3 ) [22] . The X– Hamiltonian is written The exchange interaction of the electron-hole pair with the excess electron thus acts as a Zeeman field (with sign dependence on ) on the valley pseudospin , which opens up a finite gap at the two Dirac points q X− ≡±K . X– therefore behaves like a massive Dirac fermion in the bright regions in the neighbourhood of the Dirac points (c.f. Fig. 3b ). The gap opening of the Dirac cone gives rise to a large Berry curvature with a peak value ∼ 10 4 Å 2 in the neighbourhood of q X− ≡±K , three orders of magnitude larger than that of the band edge electron in monolayer TMDCs [18] . In an in-plane electric field, X– as a charged particle will acquire a transverse velocity proportional to the Berry curvature, that is, a Hall effect. Near the Dirac points where the curvature has large value, the trion eigenstates have , hence the photon emission is circularly polarized. We note that the sign of the Berry curvature is independent of , but is correlated with the polarization of the emitted photon. The two X– configurations that will emit σ + ( σ −) photon will move towards the right (left) edge of the system (c.f. Fig. 3a ). This trion valley Hall effect may be detected by the spatially and polarization resolved PL. Typically, scattering between the states with opposite Berry curvature will suppress the Hall effect. Remarkably, such scattering is inefficient here as it requires intervalley flips of two or three electrons/holes (c.f. Fig. 3a ), and thus the valley Hall effect of X– trion is protected. The excitonic Dirac spectrum in the light cone can be mapped out by the angular resolved PL. To resolve the k -dependent splitting, a PL linewidth of about 1 meV is desirable. In monolayer MoSe 2 and WSe 2 , PL linewidth of about 5 meV has been measured at low temperature [22] , [24] . Given the much smaller radiative decay rate [19] , [34] , the measured linewidth is likely broadened due to inhomogeneous broadening and defect assisted emission [31] , and such limiting factors can be removed in cleaner systems on better substrates. Some of the predicted effects may be already observable. For example, under modest strain of 1–2%, the splitting between the two saddle points (c.f. Fig. 2 ) is already larger than the measured linewidth [22] , [24] . And for X–, the gap at the Dirac point opened by the exchange coupling is also comparable to the PL linewidth. Electrostatic screening may modify the Dirac spectrum of exciton in monolayer TMDCs. In two dimensions, the Thomas–Fermi screened Coulomb potential is of the form , where k TF is the screening wavevector. From the form of the valley-orbit coupling, it is clear that a finite screening will turn the dispersion of neutral exciton X 0 from linear to quadratic in a region of size k TF around the Dirac point, while the I remains unchanged. 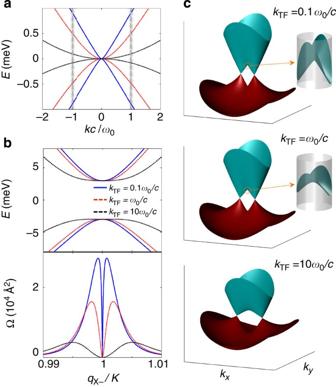Figure 4: Effect of Coulomb screening. (a) Dispersion of X0in the light cone. (b) Dispersion and Berry curvature of X–. For the blue, red and black curves, the Thomas–Fermi screening wavevectorkTF=0.1, 1 and 10, respectively, in units of ω0/c. (c) Dispersion of X0under 1% strain. For the values ofkTFconsidered, the dispersions near the pair of new Dirac points are always linear. The saddle point in the light cone changes gradually from linear dispersion forkTF≪ω0/cto quadratic one forkTF≥ω0/c. Figure 4a shows the X 0 dispersions in the light cone under different values of k TF . We consider here the regime of low doping density and relatively high temperature, where k TF is small and depends on the doping and temperature [38] , [39] . For k TF ≪ ω 0 / c , X 0 behaves like a massless chiral particle, while for k TF ≥ ω 0 / c , it will gradually cross to a massive chiral particle like the low-energy electrons in bilayer graphene. We estimate that k TF =ω 0 / c corresponds to a doping density of 10 10 cm −2 at a temperature of ∼ 30 K. Under the tensile strain, the spectrum will always split into two I =1 massless Dirac cones regardless of the value of k TF (c.f. Fig. 4c ). Nevertheless, k TF determines the dispersion of the saddle points where the two massless Dirac cones merge. The saddle point dispersion is linear for k TF ≪ ω 0 / c . For the negatively charged trion X–, we find the screening can induce a hole in the Berry curvature distribution at the Dirac point, while the peak value of the curvature remains the same order of magnitude for k TF ≤10 ω 0 / c (c.f. Fig. 4b ). Figure 4: Effect of Coulomb screening. ( a ) Dispersion of X 0 in the light cone. ( b ) Dispersion and Berry curvature of X–. For the blue, red and black curves, the Thomas–Fermi screening wavevector k TF =0.1, 1 and 10, respectively, in units of ω 0 / c . ( c ) Dispersion of X 0 under 1% strain. For the values of k TF considered, the dispersions near the pair of new Dirac points are always linear. The saddle point in the light cone changes gradually from linear dispersion for k TF ≪ ω 0 / c to quadratic one for k TF ≥ ω 0 / c . Full size image To summarize, in monolayer TMDCs, the pronounced Coulomb exchange interaction gives rise to strong valley-orbit coupling for the neutral exciton X 0 and the negatively charged trion X–. In the bright regions of the momentum space where radiative recombination can occur, these excitons offer a new venue to explore the physics of massless and massive Dirac particles. Remarkably, the energy and momentum conservation of exciton–photon interconversion allows excitons to be selectively addressed in the light cone at any specified momentum and energy, through the control of laser frequency and propagation direction. The valley optical selection rule in monolayer TMDCs also allows the optical preparation and detection of excitonic valley pseudospin [19] , [20] , [21] , [22] . These features of the exciton system in monolayer TMDCs makes possible unique opportunities to observe behaviours of Dirac particles, as compared to the electronic counterparts. Moreover, the large strain-tunable valley-orbit coupling makes monolayer TMDCs an extremely interesting playground to explore novel optoelectronic applications such as the excitonic circuit [14] and exotic quantum phenomena such as exciton condensation [12] , [13] . The ring geometry of the energy minimum and the pseudospin texture will likely lead to new structures of exciton condensates in monolayer TMDCs. How to cite this article: Yu, H. et al. Dirac cones and Dirac saddle points of bright excitons in monolayer transition metal dichalcogenides. Nat. Commun. 5:3876 doi: 10.1038/ncomms4876 (2014).